Bacterial outer membrane proteins assemble via asymmetric interactions with the BamA β-barrel The integration of β-barrel proteins into the bacterial outer membrane (OM) is catalysed by the β-barrel assembly machinery (BAM). The central BAM subunit (BamA) itself contains a β-barrel domain that is essential for OM protein biogenesis, but its mechanism of action is unknown. To elucidate its function, here we develop a method to trap a native Escherichia coli β-barrel protein bound stably to BamA at a late stage of assembly in vivo. Using disulfide-bond crosslinking, we find that the first β-strand of a laterally ‘open’ form of the BamA β-barrel forms a rigid interface with the C-terminal β-strand of the substrate. In contrast, the lipid-facing surface of the last two BamA β-strands forms weaker, conformationally heterogeneous interactions with the first β-strand of the substrate that likely represent intermediate assembly states. Based on our results, we propose that BamA promotes the membrane integration of partially folded β-barrels by a ‘swing’ mechanism. The outer membrane (OM) of Gram-negative bacteria is a key load-bearing structure [1] that is densely packed with proteins [2] . Integral outer membrane proteins (OMPs) serve multiple critical cellular functions, including nutrient uptake [3] , protein secretion [4] , [5] and adhesion [6] . Almost all of these proteins are anchored to the OM by a unique ‘β-barrel’ structure. OMP β-barrels form closed antiparallel β-sheets held together by hydrogen bonds between the first β-strand and a conserved C-terminal β-strand (the ‘β-signal’) that create a ‘β-seam’ [7] , [8] , [9] (Fig. 1a , top). The result is a highly stable amphipathic structure ranging in size from 8 to 36 β-strands with alternating hydrophobic lipid-facing and hydrophilic lumen-facing residues. Some OMPs contain separately folded extracellular or periplasmic domains or segments that are embedded inside the β-barrel [10] . Proteins that have a β-barrel architecture are also found in the OM of organelles of bacterial origin including mitochondria and chloroplasts [11] , [12] . Fig. 1 MBP−76 EspP forms a stable OMP assembly intermediate in vivo. a Top, Crystal structure of the EspP β-barrel and embedded linker (PDB id: 3slj) [42] . The β-seam between β-strand 1 (magenta) and the C-terminal β-signal stand (green, β-stand 12) is shown. Bottom, Structure of BamA derived from the cryo-EM structure of the BAM holocomplex (PDB id: 5ljo) [21] . The lateral opening between β-strand 1 (orange) and β-strands 15 (salmon) and 16 (yellow) is shown. b Primary structures of MBP−76 EspP, 76 EspP and His BamA. SS: signal sequence; TS: TwinStrepII-tag; MBP: maltose-binding protein; Pass. : passenger domain, PK: proteinase K; H: His 8 tag. Green and white triangles show the location of the surface-exposed loop cleaved by PK and the native intra-barrel cleavage site, respectively. The binding sites of antibodies/antisera used throughout this study are indicated. c Model depicting the normal assembly of 76 EspP (left) and ‘arrest-release’ assembly of MBP−76 EspP (right). During the assembly of 76 EspP, the passenger domain is secreted in a C-to N-terminal direction while the β-barrel is bound to BamA. Although the translocation of the MBP−76 EspP passenger domain is initiated properly, the MBP moiety stalls translocation and traps the β-barrel in association with BamA. Assembly can be restarted by adding PK to release an N-terminal fragment that contains the MBP moiety. d E. coli BL21(DE3) were transformed with either pMTD607/pMTD372 or pMTD826/pMTD372, and 76 EspP or MBP−76 EspP was expressed with His BamABCDE under optimised conditions (see Supplementary Fig. 1). Cells were PK-treated or mock-treated on ice. Immunoblots were then conducted using the indicated antibodies/antisera. A cross-reactive protein is denoted (*). e Reactivation of MBP−76 EspP assembly (‘arrest-release’). BL21(DE3) that expressed MBP−76 EspP and His BamABCDE were treated with PK (or mock-treated) over a 30 min time course at 25 °C. Immunoblots were then conducted using the indicated antibodies/antisera. Cross-reactive proteins are denoted (*). The fraction of the MBP−76 EspP that was completely assembled (% mature β-barrel) was calculated using the blot that was probed with αEspP βN . Representative results from at least two independent experiments are shown in d , e . Source data are provided as a Source Data file Full size image Once OMPs are translocated across the inner membrane by the Sec-translocon and maintained in an assembly-competent state by periplasmic chaperones, they are assembled and integrated into the OM in the absence of external energy inputs [13] . This is achieved by the β-barrel assembly machinery (BAM), which in E. coli is composed of a β-barrel protein (BamA) and four accessory lipoproteins (BamBCDE) that associate with the periplasmic POTRA (polypeptide transport-associated) domains of BamA [14] . Both BamA and BamD are conserved and essential for viability [15] , [16] , while bamB , bamC and bamE mutants produce variable OMP assembly defects [10] . BamA is a member of the Omp85 superfamily, a group of 16-stranded β-barrel proteins that have been implicated in both membrane protein insertion and protein secretion reactions in bacteria and organelles [17] , [18] . Despite multiple solved structures [19] , [20] , [21] , how BAM interacts with client β-barrel proteins to catalyse assembly remains the most pressing question in OMP biogenesis [13] . Two frontrunning models of OMP assembly, the ‘threading’ model (also known as the ‘budding’ model) and the ‘assisted’ model, centre on evidence that the seam between the first and last β-strands of the BamA β-barrel (β1 and β16) is structurally unstable and can open laterally (Fig. 1a , bottom). Indeed, the introduction of disulfide-bonds into BamA that prevent lateral opening of the β-barrel creates a lethal phenotype [20] , [22] and inhibits OMP assembly in vitro [21] . In the threading model, the β-strands of unfolded OMPs are threaded through the BamA β-barrel lumen and inserted sequentially into the plane of the OM through the lateral opening (the lateral ‘gate’) in BamA [22] , [23] , [24] . A hybrid-barrel is created during the assembly process that collapses when folding is complete. This model is supported by recent evidence that the mitochondrial homolog of BamA, Sam50, forms two aligned interfaces with C-terminal fragments of a mitochondrial β-barrel protein in isolated mitochondria [18] . The discovery of interactions between the C-terminal β-strand of the substrate and Sam50 β1, and the N-terminal β-strand of the substrate and Sam 50 β16, led to the proposal that insertion involves the binding of the β-signal to Sam β1, the opening and expansion of the lateral gate to accommodate an increasing number of β-hairpins, and the eventual release of the full-length protein into the lipid bilayer. The assisted model posits that the combined effects of the wedge-shape of BamA and dynamics of BamA β16 cause membrane disruption and lower the energy barrier for integration of pre-folded OMPs [24] , [25] , [26] . This model is supported by evidence that OMPs begin to fold in the periplasm prior to integration [27] , [28] , [29] , [30] , [31] , [32] , that BamA lowers the kinetic barrier for OMP insertion imposed by lipid head groups [33] , and that BamA exerts a greater stimulatory effect on the insertion of OMPs into thicker bilayers [34] . In this model, BamA is more passive, and no specific interactions form between the lateral-opening and the client OMP. Here, we sought to test these models by probing interactions between BamA and an OMP assembly intermediate in vivo. To this end, we design a method to arrest the assembly of a native β-barrel while it remains stably bound to BAM. This tool allows us to precisely map interactions between BamA and the client OMP via intermolecular disulfide-bond formation. We find that the BamA β-barrel forms two dissimilar interfaces with the assembly intermediate that effectively creates a structure that we refer to as an ‘asymmetric hybrid-barrel’. This unique structure, however, does not seem to result from the stepwise threading of β-strands of the client protein from the lumen of the BamA β-barrel into the OM via a lateral gate. Our results strongly suggest an alternative model for BamA function in which it facilitates the transfer of partially folded β-barrels from the periplasm into the OM. This model accounts for the results of previous studies but differs considerably from both the ‘threading’ and ‘assisted’ models. Design of a stable OMP assembly intermediate bound to BamA To further test the mechanism of BAM-mediated membrane integration of β-barrel proteins, we sought to obtain a detailed map of interactions between BamA and a stable OMP assembly intermediate in vivo. Because most OMPs are assembled rapidly in living cells, it is challenging to isolate a native β-barrel that is stably bound to BAM at a specific stage of assembly. To overcome this problem, we exploited the unique features of ‘autotransporters’, a class of OMPs that contain an N-terminal extracellular (‘passenger’) domain in addition to an average size 12-stranded C-terminal β-barrel domain [35] . Autotransporter β-barrel domains are not completely assembled and released from BAM until the passenger domain, which is translocated across the OM in a C- to N-terminal direction via the formation of an intra-barrel hairpin, is fully secreted [27] , [36] , [37] . Nevertheless, almost the entire passenger domain can be deleted or replaced by heterologous polypeptides without affecting β-barrel assembly [34] , [38] , [39] . Based on evidence that the translocation of fully folded heterologous polypeptides by autotransporters is often limited by their size [38] , [39] , we hypothesised that the fusion of a large protein to the passenger domain would create a molecular ‘knot-in-a-rope’ that arrests assembly after the association of the β-barrel domain with BAM and the initiation of translocation. To test this idea we fused the 40 kDa maltose-binding protein (MBP), which normally folds rapidly in the periplasm, to several N-terminally truncated versions of the E. coli O157:H7 autotransporter EspP (Fig. 1b ). We chose EspP because the two domains of the protein are separated in an autocatalytic intra-barrel cleavage reaction following the completion of β-barrel assembly [40] (Fig. 1c , left). This cleavage reaction provides an important internal control that enabled us to easily monitor the assembly status of the fusion proteins. Additionally, many aspects of the assembly of EspP have been characterised [27] , [28] , [30] , [34] , [36] , [41] and the crystal structure of its β-barrel domain has been solved [40] , [42] . Consistent with our hypothesis, we found that the MBP-EspP fusions caused assembly arrest after the fusion proteins were targeted to the OM. E. coli were transformed with a low-copy plasmid encoding TwinStrepII-tagged MBP-EspP fusions controlled by the rha promoter [43] and a second plasmid encoding BAM with a His-tagged copy of BamA controlled by an IPTG-inducible promoter [41] (Fig. 1b ). In trial experiments we tested the assembly of fusion proteins that contained passenger domain fragments (‘linkers’) of varied lengths (115, 97, 76, or 59aa) between MBP and the β-barrel domain. The absence of the cleaved β-barrel domain on immunoblots showed that none of the fusion proteins were able to assemble completely (Supplementary Fig. 1a , left). If the fusion proteins were targeted to BAM and passenger domain translocation was initiated, we predicted that the linkers would be exposed on the cell surface in a hairpin conformation and subject to cleavage by added proteinase K (PK) (Fig. 1c , right). As expected, PK digestion released a ~33 kDa C-terminal fragment corresponding to the β-barrel and a small piece of the linker from all but the smallest fusion protein (Supplementary Fig. 1a , left). PK also released multiple ~50 kD N-terminal fragments from the two largest fusion proteins that were detected on immunoblots with an anti-StrepII antibody, but only a single N-terminal fragment from the fusion containing the 76aa-linker. Furthermore, only the fusion that contains the 76aa-linker was resistant to cleavage by endogenous periplasmic proteases. This observation plus the presence of a single N-terminal PK fragment indicates that the fusion is stably trapped at a specific stage of assembly in which the folded MBP moiety remains close to the OM after it reaches BAM (Supplementary Fig. 1a , right). We therefore performed all further experiments with this fusion, which we refer to as MBP−76 EspP. Note that the final version of MBP−76 EspP also contains a surface-exposed TEV cleavage-site in the linker (between EspP residues 984/985, Supplementary Fig. 1b ) that, while not exploited in this work, is likely to be useful in future studies. Under optimised MBP−76 EspP and BAM expression conditions that we used throughout this study (Supplementary Fig. 1c ), no mature β-barrel was detected and most of the fusion protein was cleaved into a C-terminal β-barrel-containing fragment and an N-terminal MBP-containing fragment (Fig. 1d ). This observation shows that the assembly of the majority of MBP−76 EspP was stably arrested at steady-state. Under the same conditions, a control protein that lacked the MBP moiety, 76 EspP, was almost all detected as mature β-barrel due to normal rapid assembly (Fig. 1 b, d). If the assembly of MBP−76 EspP can be restarted after passenger domain translocation stalls, we expected that PK treatment would cleave the surface-exposed loop of the fusion protein, and that the subsequent release of the MBP moiety into the periplasm would facilitate the completion of assembly (Fig. 1c , right). Strikingly, after cells were incubated with PK at 25 o C, ~90% of the fusion protein was fully assembled within 10 min as indicated by the accumulation of the mature β-barrel domain (Fig. 1e ). In contrast, MBP−76 EspP in mock-treated cells remained stable (Fig. 1e ). Therefore, arrested MBP−76 EspP does not fall into a non-productive pathway, but remains in an assembly-competent state that conserves interactions with BAM that occur during normal assembly. A stable β-seam forms between BamA(β1) and MBP−76 EspP(β12) Having established a model system in which the assembly of a β-barrel protein arrests stably and reversibly, we were able to begin to precisely map interactions between the arrested MBP−76 EspP assembly intermediate and BAM subunits. Although no direct evidence exists, it has been proposed that the conserved final strand of OMPs, the β-signal, interacts with BamA during assembly [13] , [44] , [45] . Based on a recent analysis of interactions between Sam50 and truncated forms of a mitochondrial outer membrane β-barrel in isolated mitochondria [18] , we hypothesised that BamA β-strand 1 [BamA(β1)] interacts with the β-signal of MBP−76 EspP [ MBP−76 EspP(β12)]. To test this, we used solved structures of BamA [19] , [20] , [21] and the EspP β-barrel [40] , [42] as a guide to replace pairs of aligned His BamA(β1) and MBP−76 EspP(β12) residues with cysteine (Fig. 2a ). We then expressed the modified MBP−76 EspP(β12) and BAM, and assessed intermolecular proximity by disulfide-bond formation in vivo after the addition of the thiol-specific oxidiser 4-DPS. In these experiments we retained the two native cysteine residues in BamA loop 6 (C690 and C700) that normally form an intramolecular disulfide-bond [46] . We found that these residues are important for loop 6 to fold into a native conformation but do not interfere with intermolecular disulfide-bond formation (Supplementary Fig. 2 ). Fig. 2 During assembly the MBP−76 EspP(β1) β-signal forms a stable antiparallel seam with BamA(β1). a Luminal residues in BamA(β1) (orange), and luminal and lipid-facing residues in MBP−76 EspP(β12) (green and pink, respectively) are shown. Foreground strands of the MBP−76 EspP β-barrel are transparent in the zoom box. The ‘luminal’ and ‘lipid-facing’ designations are based on the orientation of the residues in solved structures (5ljo, 5d0o, and 3slj) [20] , [21] , [42] . The BamA and EspP residue numbers are based on their position in the native protein sequence. b BL21(DE3) that expressed MBP−76 EspP with single cysteine substitutions at a luminal positions in β12 and His BamABCDE with cysteine substitutions at a lumen-facing positions in His BamA(β1) were mock-treated (−) or treated with 4-DPS (+). Duplex-immunoblots were then conducted using antibodies/antisera against the N-terminus of MBP−76 EspP (αStrepII, red) and the C-terminus of His BamA/BamA (αBamA C , cyan) to monitor disulfide-bond formation between cysteine pairs in vivo. The signals are overlaid for one pair ( MBP−76 EspP N1293C / His BamA G431C , right). Non-specific bands are denoted (*). c Quantitation of disulfide-bond formation between MBP−76 EspP(β12)- His BamA(β1) cysteine pairs. Experiments were performed as in b , e (see below) except that only αStrepII was used for probing immunoblots in mock-treated (‘spontaneous’) and 4-DPS-treated cells (‘catalysed’). Bars = median, N = 4. 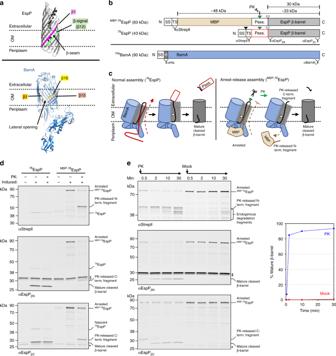Fig. 1 MBP−76EspP forms a stable OMP assembly intermediate in vivo.aTop, Crystal structure of the EspP β-barrel and embedded linker (PDB id: 3slj)42. The β-seam between β-strand 1 (magenta) and the C-terminal β-signal stand (green, β-stand 12) is shown. Bottom, Structure of BamA derived from the cryo-EM structure of the BAM holocomplex (PDB id: 5ljo)21. The lateral opening between β-strand 1 (orange) and β-strands 15 (salmon) and 16 (yellow) is shown.bPrimary structures ofMBP−76EspP,76EspP andHisBamA. SS: signal sequence; TS: TwinStrepII-tag; MBP: maltose-binding protein; Pass.: passenger domain, PK: proteinase K; H: His8tag. Green and white triangles show the location of the surface-exposed loop cleaved by PK and the native intra-barrel cleavage site, respectively. The binding sites of antibodies/antisera used throughout this study are indicated.cModel depicting the normal assembly of76EspP (left) and ‘arrest-release’ assembly ofMBP−76EspP (right). During the assembly of76EspP, the passenger domain is secreted in a C-to N-terminal direction while the β-barrel is bound to BamA. Although the translocation of theMBP−76EspP passenger domain is initiated properly, the MBP moiety stalls translocation and traps the β-barrel in association with BamA. Assembly can be restarted by adding PK to release an N-terminal fragment that contains the MBP moiety.dE. coliBL21(DE3) were transformed with either pMTD607/pMTD372 or pMTD826/pMTD372, and76EspP orMBP−76EspP was expressed withHisBamABCDE under optimised conditions (see Supplementary Fig. 1). Cells were PK-treated or mock-treated on ice. Immunoblots were then conducted using the indicated antibodies/antisera. A cross-reactive protein is denoted (*).eReactivation ofMBP−76EspP assembly (‘arrest-release’). BL21(DE3) that expressedMBP−76EspP andHisBamABCDE were treated with PK (or mock-treated) over a 30 min time course at 25 °C. Immunoblots were then conducted using the indicated antibodies/antisera. Cross-reactive proteins are denoted (*). The fraction of theMBP−76EspP that was completely assembled (% mature β-barrel) was calculated using the blot that was probed with αEspPβN. Representative results from at least two independent experiments are shown ind,e. Source data are provided as a Source Data file ANOVA and multiple comparison tests are shown in Supplementary Table 1 . d The experiments shown in b were repeated, except that misaligned lumen-facing cysteine pairs in His BamA(β1) and MBP−76 EspP(β12) were analysed. e The experiments shown in b were repeated, except that lumen-facing cysteine positions in His BamA(β1) and lipid-facing cysteine positions in MBP−76 EspP(β12) were analysed. Data are representative of at least two independent experiments for b , d and e . Source data are provided as a Source Data file Full size image Consistent with our hypothesis, we observed remarkable levels of disulfide-bond formation between aligned lumen-facing cysteines in MBP−76 EspP(β12) and His BamA(β1). After the addition of 4-DPS, 80–90% of MBP−76 EspP S1299C, MBP−76 EspP R1297C , MBP−76 EspP N1295C and MBP−76 EspP N1293C formed high molecular-weight adducts with His BamA S425C , His BamA N427C , His BamA G429C , His BamA G431C , respectively, that were detected by quantitative duplex immunoblots probed with both anti-StrepII and anti-BamA C-terminal antisera (Fig. 2b, c , Supplementary Fig. 3a ). These results, as well as the detection of appreciable levels (~5–10%) of spontaneous oxidation in the absence of 4-DPS, suggests the presence of a stable antiparallel inter-barrel interface spanning the OM when the assembly of MBP−76 EspP arrests. Importantly, the observation that the assembly of oxidised MBP−76 EspP adducts was completed upon release of the MBP-containing fragment by PK digestion and subsequent disulfide-bond reduction at 25 °C (Supplementary Fig. 4 ) confirms that the adducts remained assembly competent. We next obtained evidence that MBP−76 EspP(β12) and His BamA(β1) form a rigid, non-sliding interface during assembly. We found that distally located cysteine-pairs MBP−76 EspP N1293C / His BamA S425C and MBP−76 EspP S1299C / His BamA G431C failed to form adducts and that disulfide-bond formation was severely diminished when the residues were misaligned by only one register (Fig. 2d , Supplementary Fig. 3b ). We also did not observe significant interactions between MBP−76 EspP(β12) and His BamA(β2), MBP−76 EspP(β12) and His BamA(β15/β16), or MBP−76 EspP(β1) and His BamA(β1) (Supplementary Figs. 3d and 5 ). Because luminal residues in the mature EspP β-barrel cannot form intermolecular disulfide-bonds [40] , these results strongly suggest that both β-barrels are in an ‘open’ state when MBP−76 EspP(β12) and His BamA(β1) interact. Furthermore, when we co-expressed opposite-oriented (luminal vs. lipid-facing) cysteine-pairs to probe the flexibility and secondary structure of the interface, chemically oxidised disulfide-bond levels were typically low (~5%) and no significant spontaneous disulfide-bond was observed (Fig. 2c, e , Supplementary Fig. 3c ). The results indicate that there is considerable rigidity between MBP−76 EspP(β12) and His BamA(β1). A higher level of disulfide-bond formation between MBP−76 EspP Y1298C and His BamA S425C (28%) was observed, but is likely explained by the localisation of BamA S425 near a known flexible-hinge between the BamA β-barrel and periplasmic POTRA domains [47] . A conformationally diverse second inter-barrel interface A recent examination of interactions between Sam50 and fragments of mitochondrial outer membrane β-barrels showed that a potentially strong second interface forms between the final β-strand of Sam50 [Sam50(β16)] and the N-terminal β-strand of the client, and suggested that an expanding β-sheet enters the OM via the lumen of Sam50 [18] . To determine if a similar second interface is formed between inward-facing residues of BamA and assembly-arrested MBP−76 EspP, we introduced cysteines into luminal positions of His BamA(β16) and both lumen- and lipid-facing positions in MBP−76 EspP(β1) (Fig. 3a ). As in our analysis of the MBP−76 EspP(β12)- His BamA(β1) interface, we co-expressed cysteine pairs that we posited would be similarly aligned and oriented. However, the luminal residues MBP−76 EspP R1044C , MBP−76 EspP W1042C , and MBP−76 EspP G1040C displayed only low levels of chemically-induced disulfide-bond formation (1–5%) with His BamA N805C , His BamA G807C and His BamA T809C , respectively, based on quantitative immunoblot analysis (Fig. 3b, c , Supplementary Fig. 6a , b). Even lower levels of interaction were detected when the lipid-facing cysteines MBP−76 EspP I1045C , MBP−76 EspP A1043C and MBP−76 EspP A1041C were paired with His BamA N805C , His BamA G807C and His BamA T809C , respectively, or when any of the six MBP−76 EspP(β1) cysteines were paired in any combination with luminal cysteines in His BamA(β16) (Supplementary Fig. 6c–e ). Despite the low levels of disulfide-bond formation, His BamA T809C consistently produced higher adduct levels regardless of the cysteine location in MBP−76 EspP(β1). This observation implies significant structural promiscuity and is in line with previous reports of dynamicity and kink formation in BamA(β16) [20] , [21] , [25] , [47] . Nevertheless, the results strongly suggest that BamA does not form two matching interfaces with client proteins. Fig. 3 MBP−76 EspP(β1) cysteines bond weakly with luminal-facing cysteines in BamA(β16). a Left, view of BamA showing β-strand 16 (yellow) and lumen-facing residue N805. Note that the last several residues of BamA(β16) are not resolved in available structures. Right, view of MBP−76 EspP(β1) showing lipid-facing (magenta) and lumen-facing (orange) residues. Foreground strands of the EspP β-barrel (including β12, green) are transparent. b BL21(DE3) that expressed MBP−76 EspP with a cysteine substitution at a luminal position in β1 and His BamABCDE with a cysteine substitution at a luminal position in His BamA(β16) were mock-treated (−) or treated with 4-DPS (+). Duplex-immunoblots were then conducted using antibodies/antisera against the C-terminus of MBP−76 EspP (αEspP βC ) and the N-terminus of His BamA (αHis) to monitor disulfide-bond formation between cysteine pairs in vivo. Non-specific bands are denoted (*). Data are representative of at least two independent experiments. c Quantitation of disulfide-bond formation between MBP−76 EspP(β1)- His BamA(β16) cysteine-pairs in cells that were 4-DPS-treated. Experiments were performed as in b except that only αStrepII was used for probing immunoblots. Bars = median, N = 4. 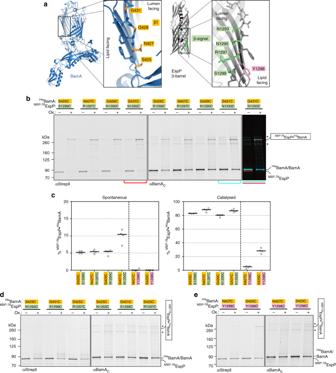Fig. 2 During assembly theMBP−76EspP(β1) β-signal forms a stable antiparallel seam with BamA(β1).aLuminal residues in BamA(β1) (orange), and luminal and lipid-facing residues inMBP−76EspP(β12) (green and pink, respectively) are shown. Foreground strands of theMBP−76EspP β-barrel are transparent in the zoom box. The ‘luminal’ and ‘lipid-facing’ designations are based on the orientation of the residues in solved structures (5ljo, 5d0o, and 3slj)20,21,42. The BamA and EspP residue numbers are based on their position in the native protein sequence.bBL21(DE3) that expressedMBP−76EspP with single cysteine substitutions at a luminal positions in β12 andHisBamABCDE with cysteine substitutions at a lumen-facing positions inHisBamA(β1) were mock-treated (−) or treated with 4-DPS (+). Duplex-immunoblots were then conducted using antibodies/antisera against the N-terminus ofMBP−76EspP (αStrepII, red) and the C-terminus ofHisBamA/BamA (αBamAC, cyan) to monitor disulfide-bond formation between cysteine pairs in vivo. The signals are overlaid for one pair (MBP−76EspPN1293C/HisBamAG431C, right). Non-specific bands are denoted (*).cQuantitation of disulfide-bond formation betweenMBP−76EspP(β12)-HisBamA(β1) cysteine pairs. Experiments were performed as inb,e(see below) except that only αStrepII was used for probing immunoblots in mock-treated (‘spontaneous’) and 4-DPS-treated cells (‘catalysed’). Bars = median,N= 4. ANOVA and multiple comparison tests are shown in Supplementary Table1.dThe experiments shown inbwere repeated, except that misaligned lumen-facing cysteine pairs inHisBamA(β1) andMBP−76EspP(β12) were analysed.eThe experiments shown inbwere repeated, except that lumen-facing cysteine positions inHisBamA(β1) and lipid-facing cysteine positions inMBP−76EspP(β12) were analysed. Data are representative of at least two independent experiments forb,dande. Source data are provided as a Source Data file ANOVA and multiple comparison tests are shown in Supplementary Table 2 . Source data are provided as a Source Data file Full size image A close inspection of the BAM cryo-EM structure [21] shows that when BamA is in a ‘lateral-open’ state, BamA(β15) and BamA(β16) are twisted downward towards the periplasm and curled inward towards the β-barrel lumen. We hypothesised that this unusual conformation might present a unique ‘outward-facing’ surface that is proximal to the first β-strand of client β-barrels. To test this idea, we substituted cysteine for F785 and I806, two outward-facing amino acids in His BamA(β15) and His BamA(β16), respectively, that are predicted to reside at a similar membrane depth, and paired them with MBP−76 EspP(β1) cysteine substitutions that span the OM (Fig. 4a ). A cysteine was also substituted for His BamA V784 to provide a lumen-facing control. Fig. 4 Bonding of MBP−76 EspP(β1) cysteines with lipid-facing cysteines in BamA(β15/16). a Left, view of outward-facing residues I806 in BamA(β16) (yellow) and F785 in BamA(β15) (salmon). Right, view of MBP−76 EspP(β1) showing lipid-facing (magenta) and luminal (orange) residues. Residue S1047 is situated at the interface between the outer leaflet of the OM and the extracellular milieu [54] and is the last membrane embedded residue of β1. b , d BL21(DE3) that expressed MBP−76 EspP with a single cysteine substitution in β1 and His BamABCDE with a His Bam I806C ( b ) or His BamA F785C ( d ) substitution were mock-treated (−) or treated with 4-DPS (+). Duplex-immunoblots were then conducted using antibodies/antisera against the N-terminus and C-terminus of MBP−76 EspP (αStrepII or αEspP βC ) and His BamA (αHis or αBamA C ) to monitor disulfide-bond formation between cysteine pairs in vivo. Non-specific bands are denoted (*). Data are representative of at least two independent experiments. c , e Quantitation of disulfide-bond formation between MBP−76 EspP(β1) and His Bam I806C ( c ) or His BamA F785C ( e ) cysteine pairs in 4-DPS-treated cells. Experiments were performed as in b , d except that only αStrepII was used for probing immunoblots. Bars = median, N = 4. ANOVA and multiple comparison tests are shown in Supplementary Tables 3 and 4 . Source data are provided as a Source Data file Full size image Consistent with our hypothesis, we observed a significant level of 4-DPS-mediated disulfide-bond formation (typically ~10–20%) between His BamA F785C and all of the MBP−76 EspP(β1) cysteine residues we tested (Fig. 4b, c ; Supplementary Fig. 7 a, c). There was no clear dependence on the orientation of the MBP−76 EspP(β1) cysteine residue. Interestingly, cysteines in the middle of the OM spanning segment ( MBP−76 EspP A1043C and MBP−76 EspP R1044C ) formed adducts considerably less efficiently than adjacent cysteines. This observation suggests that MBP−76 EspP(β1) occupies at least two conformational states relative to His BamA(β15). In contrast, none of the MBP−76 EspP(β1) positions formed adducts with His BamA V784C (Supplementary Fig. 7d ). Thus the outward-facing surface rather than the luminal side of His BamA(β15) is in proximity to MBP−76 EspP(β1). Significant, but less efficient chemically oxidised disulfide-bond formation was also observed between MBP−76 EspP(β1) cysteines and His BamA I806C (typically ~5–15%) that was likewise orientation-independent (Fig. 4d, e , Supplementary Fig. 7b, c ). Because we observed consistently lower interactions between MBP−76 EspP(β1)/ His BamA(β16) pairs than between MBP−76 EspP(β12)/ His BamA(β1) pairs, we checked if any of the MBP−76 EspP(β1) cysteine mutants affected protein biogenesis. We found that the linkers of all but MBP−76 EspP G1040C and MBP−76 EspP W1042C (which contain substitutions at conserved but uncharacterised autotransporter residues) were protease sensitive and therefore properly exposed on the cell surface (Supplementary Fig. 7e ). Given that prolonged periplasmic exposure of the EspP β-barrel leads to its degradation, however, the stability of the two mutant proteins, in addition to the consistency of the overall disulfide-bonding pattern, indicate that the G1040C and W1042C substitutions do not affect the engagement of MBP−76 EspP by BAM. Taken together, these data provide clear evidence for the formation of discrete, heterogeneous interactions between the outward-facing surface of BamA(β15/β16) and MBP−76 EspP(β1) that were not observed in the analysis of Sam50 function [18] . Because our analysis of F785 interactions strongly suggested that the outward-facing surface of BamA(β15) creates a unique interface with MBP−76 EspP(β1), we sought to investigate BamA(β15) interactions at positions closer to the periplasmic side of the OM. Perhaps because L783 and P782 are essential for function, we could not introduce cysteine substitutions at these positions. However, we were able to obtain His BamA G781C and to assess the formation of disulfide-bonds between this residue and the aforementioned MBP−76 EspP(β1) cysteine substitutions (Fig. 5a ). Upon the addition of oxidiser most cysteine-pairs formed a modest level of disulfide-bonded adducts (~10%) that was similar to the levels observed in the analysis of His BamA F785C (Fig. 5b, c , Supplementary Fig. 8 ). However, the level of disulfide-bond formation between the lipid-facing MBP−76 EspP A1043C residue and His BamA G781C was considerably higher (42%) than that formed between any other MBP−76 EspP(β1)/ His BamA(β15/β16) cysteine-pair (Fig. 5b, c ). The results suggest that MBP−76 EspP A1043C and His BamA G781C are in close proximity in the most probable of multiple conformational states that can be occupied by MBP−76 EspP(β1) and the C-terminus of BamA when the assembly of MBP−76 EspP stalls. Importantly, the interaction of A1043C, which is located near the middle of the OM spanning segment of MBP−76 EspP(β1), with His BamA G781C , which is located close to the periplasm, strongly suggests that MBP−76 EspP(β1) is partially in the periplasm and not stably integrated into the OM in this conformational state. Fig. 5 Strong bond between a mid-strand MBP−76 EspP(β1) cysteine and a periplasmic-proximal BamA(β15) cysteine. 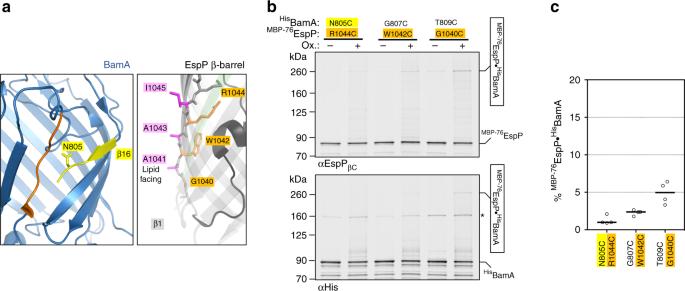Fig. 3 MBP−76EspP(β1) cysteines bond weakly with luminal-facing cysteines in BamA(β16).aLeft, view of BamA showing β-strand 16 (yellow) and lumen-facing residue N805. Note that the last several residues of BamA(β16) are not resolved in available structures. Right, view ofMBP−76EspP(β1) showing lipid-facing (magenta) and lumen-facing (orange) residues. Foreground strands of the EspP β-barrel (including β12, green) are transparent.bBL21(DE3) that expressedMBP−76EspP with a cysteine substitution at a luminal position in β1 andHisBamABCDE with a cysteine substitution at a luminal position inHisBamA(β16) were mock-treated (−) or treated with 4-DPS (+). Duplex-immunoblots were then conducted using antibodies/antisera against the C-terminus ofMBP−76EspP (αEspPβC) and the N-terminus ofHisBamA (αHis) to monitor disulfide-bond formation between cysteine pairs in vivo. Non-specific bands are denoted (*). Data are representative of at least two independent experiments.cQuantitation of disulfide-bond formation betweenMBP−76EspP(β1)-HisBamA(β16) cysteine-pairs in cells that were 4-DPS-treated. Experiments were performed as inbexcept that only αStrepII was used for probing immunoblots. Bars = median,N= 4. ANOVA and multiple comparison tests are shown in Supplementary Table2. Source data are provided as a Source Data file a Left, view of periplasmic-proximal BamA β-strand 15 residue G781 (red) in the lateral opening. Right, view of MBP−76 EspP(β1) showing lipid-facing (magenta) and luminal (orange) residues. b BL21(DE3) that expressed MBP−76 EspP with a single cysteine substitution in β1 and His BamABCDE with the His BamA G781C substitution were mock-treated (−) or treated with 4-DPS (+). Duplex-immunoblots were then conducted using antibodies/antisera against the N-terminus of MBP−76 EspP (αStrep II) and the C-terminus of His BamA (αBamA C ) to monitor disulfide-bond formation between cysteine pairs in vivo. Non-specific bands are denoted (*). 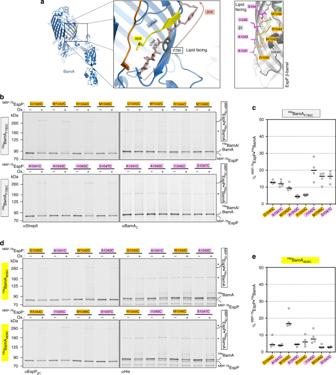Fig. 4 Bonding ofMBP−76EspP(β1) cysteines with lipid-facing cysteines in BamA(β15/16).aLeft, view of outward-facing residues I806 in BamA(β16) (yellow) and F785 in BamA(β15) (salmon). Right, view ofMBP−76EspP(β1) showing lipid-facing (magenta) and luminal (orange) residues. Residue S1047 is situated at the interface between the outer leaflet of the OM and the extracellular milieu54and is the last membrane embedded residue of β1.b,dBL21(DE3) that expressedMBP−76EspP with a single cysteine substitution in β1 andHisBamABCDE with aHisBamI806C(b) orHisBamAF785C(d) substitution were mock-treated (−) or treated with 4-DPS (+). Duplex-immunoblots were then conducted using antibodies/antisera against the N-terminus and C-terminus ofMBP−76EspP (αStrepII or αEspPβC) andHisBamA (αHis or αBamAC) to monitor disulfide-bond formation between cysteine pairs in vivo. Non-specific bands are denoted (*). Data are representative of at least two independent experiments.c,eQuantitation of disulfide-bond formation betweenMBP−76EspP(β1) andHisBamI806C(c) orHisBamAF785C(e) cysteine pairs in 4-DPS-treated cells. Experiments were performed as inb,dexcept that only αStrepII was used for probing immunoblots. Bars = median,N= 4. ANOVA and multiple comparison tests are shown in Supplementary Tables3and4. Source data are provided as a Source Data file Data are representative of at least two independent experiments. c Quantitation of disulfide-bond formation between MBP−76 EspP(β1) and His BamA G781C cysteine pairs in mock-treated cells (‘spontaneous’) and 4-DPS-treated cells (‘catalysed’). Experiments were performed as in b , except that only αStrepII was used for probing immunoblots. Bars = median, N = 4. 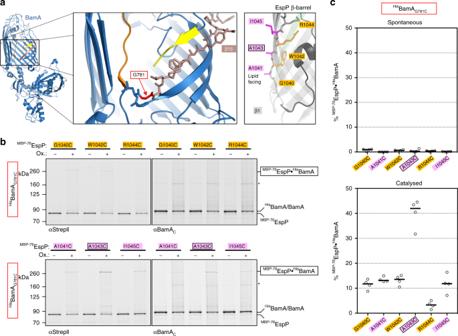Fig. 5 Strong bond between a mid-strandMBP−76EspP(β1) cysteine and a periplasmic-proximal BamA(β15) cysteine.aLeft, view of periplasmic-proximal BamA β-strand 15 residue G781 (red) in the lateral opening. Right, view ofMBP−76EspP(β1) showing lipid-facing (magenta) and luminal (orange) residues.bBL21(DE3) that expressedMBP−76EspP with a single cysteine substitution in β1 andHisBamABCDE with theHisBamAG781Csubstitution were mock-treated (−) or treated with 4-DPS (+). Duplex-immunoblots were then conducted using antibodies/antisera against the N-terminus ofMBP−76EspP (αStrep II) and the C-terminus ofHisBamA (αBamAC) to monitor disulfide-bond formation between cysteine pairs in vivo. Non-specific bands are denoted (*). Data are representative of at least two independent experiments.cQuantitation of disulfide-bond formation betweenMBP−76EspP(β1) andHisBamAG781Ccysteine pairs in mock-treated cells (‘spontaneous’) and 4-DPS-treated cells (‘catalysed’). Experiments were performed as inb, except that only αStrepII was used for probing immunoblots. Bars = median,N= 4. ANOVA and multiple comparison tests are shown in Supplementary Table5. Source data are provided as a Source Data file ANOVA and multiple comparison tests are shown in Supplementary Table 5 . Source data are provided as a Source Data file Full size image The two MBP−76 EspP-BamA interfaces exhibit distinct features Several observations suggested that when the assembly of MBP−76 EspP is arrested, it forms two very different barrel-barrel interfaces with BamA. The interaction of BamA(β1) and the MBP−76 EspP β-signal created a rigid, antiparallel, non-sliding inter-barrel β-seam. The formation of disulfide-bonds even in the absence of an oxidant attested to the high stability of this interaction. In contrast, MBP−76 EspP(β1) did not form an analogous interface with His BamA(β16) but rather weaker, more flexible, interactions with outward-facing positions in both His BamA(β15) and His BamA(β16) that were dependent on the addition of an oxidant. Because no single placement of MBP−76 EspP(β1) relative to His BamA(β15/16) can account for all of the disulfide-bonds we observed (Fig. 6a ), it is likely that multiple conformations that reflect snapshots of different stages of assembly existed. Fig. 6 Distinct properties of the two interfaces formed between MBP−76 EspP and BamA. a Models of interactions between MBP−76 EspP(β1) and BamA(β15/β16) based on disulfide-bond formation data in Figs. 4 and 5 . MBP- 76 EspP(β1) (black), and antiparallel BamA β15 (salmon) and β16 (yellow), are shown as arrows. The BamA β-strands are tilted to match their orientation in solved structures. Key residues are represented by coloured circles. Cysteine-pairs that formed disulfide-bonds at a median level of 10–20% are denoted by blue lines while levels above 40% are denoted by a blue oval. Although no single model can completely explain the observed disulfide-bond patterns, placement of MBP− 76 EspP(β1) in the two orientations that are shown accounts for most of the data. b BL21(DE3) that expressed MBP−76 EspP S1299C / His BamA S425C (blue) or MBP−76 EspP A1043C / His BamA G781C (red) pairs were treated with 4-DPS on ice over a 90 min time course and the kinetics of disulfiide-bond formation was quantitated from immunoblots probed with αStrepII. The MBP−76 EspP S1299C / His BamA S425C data could not be fit to a single-step binding curve (R 2 = −14.94), while the MBP−76 EspP A1043C / His BamA G781C data could be fit (R 2 = 0.98, K = 0.038 ± 0.004 min −1 , half-time = 18.2 min). Points = mean ± standard error, N = 3. c BL21(DE3) that expressed MBP−76 EspP S1299C / His BamA S425C or MBP−76 EspP A1043C / His BamA G781C pairs were treated with 4-DPS. Cell lysates were either unheated (0 °C) or heated (99 °C) and proteins were resolved by cold SDS-PAGE. Duplex-immunoblots were then conducted using αEspP βC /αHis or αStrepII/αBamA C antisera/antibodies. Right, image analysis of the boxed regions of the blots was performed using Fiji software and false colouring. Horizontal average intensity plots (arbitrary values) are shown, and distinct peaks are numbered. Representative results from at least two independent experiments are shown. Source data are provided as a Source Data file Full size image To further examine the asymmetry between the two barrel-barrel interfaces, we compared the kinetics of disulfide-bond formation between pairs MBP−76 EspP S1299C / His BamA S425C (representing the MBP−76 EspP(β12- His BamA(β1) interface) and MBP−76 EspP A1043C / His BamA G781C (representing a major conformer of the MBP−76 EspP(β1)- His BamA (β15/β16) interface). A large fraction of the MBP−76 EspP S1299C / His BamA S425C pair formed adducts extremely rapidly and plateaued almost immediately, while cells that expressed MBP−76 EspP A1043C / His BamA G781C displayed a slow accumulation of adducts during an extended incubation period before plateauing at a much lower level (Fig. 6b , Supplementary Fig. 9a , b). The results show a clear difference in the association stabilities between the two inter-barrel interfaces and presumably reflect a difference in local conformational flexibility. The difference in plateaus also provides evidence that when only interactions between His BamA G781C and MBP−76 EspP A1043C are monitored, alternate conformations between MBP−76 EspP(β1) and the C-terminus of His BamA remain unaccounted for. To obtain direct evidence that the two inter-barrel interfaces have distinct conformational properties, we exploited the remarkable ability of folded β-barrels to resist SDS denaturation in the absence of heat and migrate relatively rapidly on SDS-PAGE. As in the previous experiment, we expressed either MBP−76 EspP S1299C / His BamA S425C or MBP−76 EspP A1043C / His BamA G781C pairs and catalysed disulfide-bond formation with 4-DPS. Cell lysates were then kept on ice or boiled, and proteins were resolved by SDS-PAGE at 0–4 °C. Interestingly, the unheated MBP−76 EspP S1299C - His BamA S425C adduct was detected on duplex immunoblots as at least three discrete fast-migrating species that likely represent distinct conformational states (Fig. 6c , top). Identical results were obtained when the experiment was repeated with another MBP−76 EspP(β12)- His BamA(β1) pair ( MBP−76 EspP N1293C / His BamA G431C ) (Supplementary Fig. 9b, c ). The unheated MBP−76 EspP A1043C - His BamA G781C - adduct, however, was detected as only a single fast-migrating species (Fig. 6c , bottom). Consistent with the results of previous experiments, these results suggest that when the stable MBP−76 EspP(β12)- His BamA(β1) inter-barrel β-seam is tethered by a disulfide-bond, the opposing MBP−76 EspP(β1)-BamA C-terminus interface remains free to adopt multiple intermediate conformations. Conversely, when the MBP−76 EspP(β1)- His BamA(β15) interface is locked, only one conformation is observed because the opposing inter-barrel β-seam exists as a single stable state. In this study we describe a structure-guided interaction map of BamA bound to an OMP assembly intermediate in vivo with disulfide-bond resolution. To perform our analysis, we first engineered a fusion protein in which an MBP moiety arrests the translocation of an autotransporter passenger domain and thereby traps the β-barrel in a stable, incompletely assembled state. After validating MBP−76 EspP as an assembly intermediate by showing that the arrest of assembly is reversible, we pinpointed positions in BamA and MBP−76 EspP β-barrels that are in close proximity by monitoring intermolecular disulfide-bond formation after the addition of an oxidant. We found that the two proteins interact via two distinct interfaces that create an asymmetric hybrid-barrel. On one side, the EspP β-signal formed a rigid antiparallel inter-barrel β-seam with BamA(β1). This observation rules out an ‘assisted’ model in which BamA catalyses assembly simply by perturbing the lipid bilayer. Unexpectedly, no analogous interface between BamA(β16) and MBP−76 EspP(β1) was observed. Instead, we identified diverse, relatively weak interactions between the outward-facing surface of BamA(β15/β16) and MBP−76 EspP(β1) that indicated the presence of multiple conformations. Remarkably, in the most common conformer the middle of the MBP−76 EspP(β1) transmembrane segment was positioned near the most periplasmic-proximal position of BamA(β15). In this state, part of the EspP β-barrel presumably remained in the periplasm. Finally, an analysis of disulfide-bond formation kinetics and mobility states on SDS-PAGE provided direct evidence that one inter-barrel interface is stable, while the other is conformationally heterogeneous. Although hybrid-barrel formation and an analogous interaction between Sam50(β1) and the β-signal of client proteins was also recently reported in an examination of interactions between Sam50 and C-terminal fragments of mitochondrial β-barrels [18] , our results differ from those of the previous study in several critical respects. First, the previous study reported a potentially strong interface between Sam50(β16) and the N-terminal β-strand of the client that we did not observe in our analysis of the interaction of BamA and MBP−76 EspP. Second, a predominant conformational state in which the first β-strand of an incoming β-barrel does not appear to be fully integrated into the OM ( MBP−76 EspP A1043C - His BamA G781C ) was not identified in the Sam50 study. Most significantly, while we observed disulfide-bond formation between MBP−76 EspP(β1) and the outward-facing surface of BamA(β15/16), chemical crosslinking of N-terminal residues of mitochondrial β-barrel fragments to luminal residues of Sam50(β15) and an internal loop of Sam50 was observed in the previous study. Those results provided evidence for a model involving initial threading of unfolded β-barrels into the Sam50 lumen, progressive folding between the two sides of an open Sam50 lateral-gate, and release of the full-length protein into the lipid bilayer [18] . Similar models for OMP assembly that posit the stepwise formation of a hybrid-barrel within the plane of the OM have been proposed based on the crystal structures of BamA [24] and TamA [48] , another member of the Omp85 family. There are several possible explanations for the discrepancies between our study and the Sam50 study. It is conceivable that the use of β-barrel fragments in the Sam50 study captured an earlier stage of the assembly process than we observed through the use of a complete β-barrel. Alternatively, N-terminally truncated mitochondrial β-barrels might interact differently with Sam50 than native clients in vivo. An especially intriguing possibility, particularly in light of the functional diversity of members of the Omp85 superfamily [5] , [17] , is that the catalytic mechanisms of BamA and Sam50 have diverged. Indeed, S. cerevisiae Sam50 and E. coli BamA share only 21% sequence similarity, have a different number of POTRA domains, function in dissimilar membrane environments, and form complexes with unrelated accessory proteins that have opposite membrane topologies [11] . Furthermore, Sam50 and BamA may catalyse the assembly of client proteins that have distinct folding requirements. For instance, bacterial OMPs are profoundly structurally diverse and contain an even number of β-strands that necessitates the formation of an antiparallel β-seam, while mitochondrial β-barrels (besides Sam50) are all members of a single family of 19-stranded proteins that have a parallel β-seam [11] , [49] . Importantly, if the assembly mechanisms used by Sam50 and BamA have diverged, it might be possible to design antibiotics that target BamA [50] but that do not cause mitochondrial toxicity. Regardless of the reason that disparate results were obtained in the two studies, we propose that BamA functions by actively integrating client proteins into the OM from the periplasm via a ‘swing’ mechanism rather than progressively threading them through a lateral gate. In this model, the β-signal of a partially folded client protein forms a transiently stable interaction with BamA(β1) that creates an inter-barrel β-seam (Fig. 7 , stage i; Supplementary Video 1 ). The inter-barrel β-seam maintains the association between the two barrels while BamA acts as a molecular hinge that allows the N-terminus of the client β-barrel to move along the outward-facing surface of its C-terminal strands and integrate into the OM through a swinging action (Fig. 7 , stage ii). Although we cannot order a series of intermediate conformations from our steady-state data, it seems likely that the diverse interactions that we observed between MBP−76 EspP(β1) and lipid-exposed residues of BamA(β15/β16) represent assembly snapshots of the partially folded OMP moving along the outward-facing surface of BamA into the plane of the OM. The strong MBP−76 EspP A1043C - His BamA G781C interaction (which in itself provides clear evidence that the β-strands do not simply partition into the lipid bilayer through a lateral-gate) presumably corresponds to an early state in which much of the client is still positioned in the periplasm. In a final step, the client is released from BamA into the lipid bilayer as a fully assembled β-barrel (Fig. 7 , stage iii). We speculate that the asymmetry helps complete assembly by promoting the energetically favourable closure of the client β-barrel and restoration of the BamA ground state through a β-signal exchange (Fig. 7 , stage iv). Fig. 7 Model of bacterial outer membrane protein assembly. Red arrows indicate possible conformational changes. After an OMP (grey) is targeted to the OM, it interacts with the BamA β-barrel (blue). Initially the C-terminal β-strand of the OMP (β-signal, green) forms a β-seam with BamA β1 (orange) to create an asymmetric hybrid barrel (i). It is not yet clear if the OMP begins to fold before or after the formation of this interface. Subsequently the first β-strand of the OMP (magenta) forms a low stability interface with the outward-facing surface of BamA β15/16 (salmon/yellow) (ii). A large-scale movement of the OMP into the membrane (‘swing’) is aided by the rotation of BamA β1-β8, the perturbation of the lipid bilayer by the wedge-shape of the BamA β-barrel, and the dynamicity of β16. The asymmetry between the two interfaces favours the closure of the client β-barrel (iii) and its release into the lipid bilayer in a native conformation (iv). Our results suggest that a loop of the MBP−76 EspP passenger domain is exposed on the cell surface prior to most of the swinging action Full size image The results of numerous previous studies on OMP biogenesis are consistent with a ‘swing’ model for BamA function. First and foremost, there is now considerable evidence from in vivo studies on EspP, trimeric adhesins and the LPS transporter complex LptDE that OMPs begin to fold prior to their integration into the OM [27] , [28] , [29] , [30] , [31] , [32] and are therefore unlikely to be inserted by progressive threading. Many of the results suggest that folding begins in the periplasm or is promoted by interactions with the BAM lipoproteins or the BamA POTRA domains that precede interactions with the BamA β-barrel. As suggested in a recently proposed ‘elongation’ model, however, it is conceivable that the initial association of the β-signal with BamA(β1) nucleates subsequent C- to N-terminal folding on the periplasmic side of the OM [10] . Second, evidence that the effect of lipid-facing arginine residues on OMP biogenesis is highly dependent on membrane depth is consistent with the notion that charged groups hinder productive passage through a hydrophobic environment [51] . Structural studies also support a ‘swing’ model. Solved structures of BAM show that the transition between the ‘closed’ and ‘open’ states of the BamA β-barrel involves a remarkable scissor-like 45°–65° rotation of BamA(β1–β8) [19] , [20] that could represent the hinge mechanism for a major swinging action of client OMPs. There is also substantial evidence that the wedge-shaped aromatic-girdle of BamA and the highly dynamic properties of BamA(β16) promote membrane thinning and disorder near the lateral opening [24] , [25] , [26] , [47] . This membrane perturbation would potentially drive the swinging movement of partially folded β-barrels into the OM by lowering the energy barrier for integration and by promoting hydrophobic interactions between their outer surface and membrane lipids. Finally, our model fits well with recent bioinformatic evidence that the C-terminal half of OMPs is especially well conserved [52] . We speculate that the need to form an asymmetric hybrid-barrel during assembly constrains the C-terminal sequences of OMPs but provides the freedom for evolution through N-terminal modifications [52] . 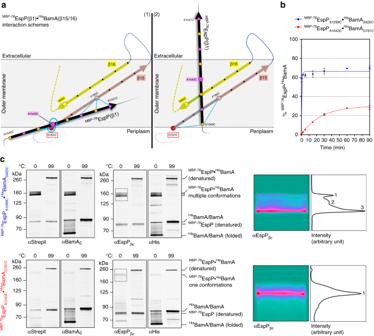Fig. 6 Distinct properties of the two interfaces formed betweenMBP−76EspP and BamA.aModels of interactions betweenMBP−76EspP(β1) and BamA(β15/β16) based on disulfide-bond formation data in Figs.4and5.MBP-76EspP(β1) (black), and antiparallel BamA β15 (salmon) and β16 (yellow), are shown as arrows. The BamA β-strands are tilted to match their orientation in solved structures. Key residues are represented by coloured circles. Cysteine-pairs that formed disulfide-bonds at a median level of 10–20% are denoted by blue lines while levels above 40% are denoted by a blue oval. Although no single model can completely explain the observed disulfide-bond patterns, placement ofMBP−76EspP(β1) in the two orientations that are shown accounts for most of the data.bBL21(DE3) that expressedMBP−76EspPS1299C/HisBamAS425C(blue) orMBP−76EspPA1043C/HisBamAG781C(red) pairs were treated with 4-DPS on ice over a 90 min time course and the kinetics of disulfiide-bond formation was quantitated from immunoblots probed with αStrepII. TheMBP−76EspPS1299C/HisBamAS425Cdata could not be fit to a single-step binding curve (R2= −14.94), while theMBP−76EspPA1043C/HisBamAG781Cdata could be fit (R2= 0.98, K = 0.038 ± 0.004 min−1, half-time = 18.2 min). Points = mean ± standard error,N= 3.cBL21(DE3) that expressedMBP−76EspPS1299C/HisBamAS425CorMBP−76EspPA1043C/HisBamAG781Cpairs were treated with 4-DPS. Cell lysates were either unheated (0 °C) or heated (99 °C) and proteins were resolved by cold SDS-PAGE. Duplex-immunoblots were then conducted using αEspPβC/αHis or αStrepII/αBamACantisera/antibodies. Right, image analysis of the boxed regions of the blots was performed using Fiji software and false colouring. Horizontal average intensity plots (arbitrary values) are shown, and distinct peaks are numbered. Representative results from at least two independent experiments are shown. Source data are provided as a Source Data file Plasmid construction The plasmids that were used in our experiments are listed in Supplementary Table 6 . 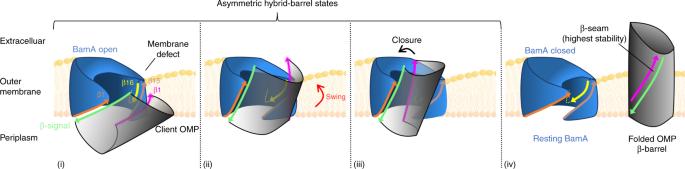Fig. 7 Model of bacterial outer membrane protein assembly. Red arrows indicate possible conformational changes. After an OMP (grey) is targeted to the OM, it interacts with the BamA β-barrel (blue). Initially the C-terminal β-strand of the OMP (β-signal, green) forms a β-seam with BamA β1 (orange) to create an asymmetric hybrid barrel (i). It is not yet clear if the OMP begins to fold before or after the formation of this interface. Subsequently the first β-strand of the OMP (magenta) forms a low stability interface with the outward-facing surface of BamA β15/16 (salmon/yellow) (ii). A large-scale movement of the OMP into the membrane (‘swing’) is aided by the rotation of BamA β1-β8, the perturbation of the lipid bilayer by the wedge-shape of the BamA β-barrel, and the dynamicity of β16. The asymmetry between the two interfaces favours the closure of the client β-barrel (iii) and its release into the lipid bilayer in a native conformation (iv). Our results suggest that a loop of theMBP−76EspP passenger domain is exposed on the cell surface prior to most of the swinging action Oligonucleotide primers and dsDNA fragments that were used in plasmid construction are listed in Supplementary Table 7 . To construct pMTD321, a plasmid that encodes an MBP fusion to the EspP β-barrel with a 115aa-linker, a DNA fragment encoding malE was PCR amplified using primers Mal.Eag(+)/Mal.Eag(−) and pMAL-p2x as a template, digested with EagI, and ligated into the EagI site of pJH64 [53] to create pJH64:: malE . The open reading frame of the fusion protein was then PCR amplified using primers mtd1/pTRC 399 R and pJH64:: malE as a template, digested with NdeI and HindIII, and sub-cloned into similarly digested pWK1 [38] , a derivative of the rhamnose-inducible plasmid pSCrhaB2 [43] . Finally, the resulting plasmid was PCR amplified with primers mtd96/mtd97 and mixed with dsDNA fragment mtd95 to attach a TwinStrepII-tag to the fusion protein via Gibson assembly. To construct plasmids that encode MBP fusions to the EspP β-barrel with 97, 76, or 59aa-linkers (pMTD501, pMTD502 and pMTD610, respectively), pMTD321 was PCR amplified using primers mtd145/mtd146, mtd145/mtd147, or mtd145/164, respectively, digested with BamHI, and re-circularised. To make pMTD521 and pMTD607 (pRha MBP−76 EspP), which encode an MBP fusion to the EspP β-barrel with a 76aa-linker and a TEV cleavage site between EspP residues 974/975 or 984/985, respectively, pMTD502 was PCR amplified using primers mtd135/136 or mtd160/161 and assembled with mtd137 or mtd159 dsDNA fragments (encoding TEV cleavage sites). Plasmid pMTD826, which encodes 76 EspP, was generated by first introducing a second BamHI site into pMTD607 using primers mtd186/187 together with the QuikChange II Site-Directed Mutagenesis Kit (Agilent). The resulting plasmid (pMTD798) was then digested with BamHI and re-circularised. To construct pMTD372 (pTrc99a:: His8 bamABCDE ), pJH114 [34] was PCR amplified using primers mtd102/mtd103 and assembled with dsDNA fragment mtd101 (encoding a His8 tag). The resulting plasmid (pMTD366) was subsequently mutagenised using primers mtd104/mtd105 to re-introduce the native bamE stop codon. Cysteine substitution mutations were introduced into pMTD372 and pMTD607 by site-directed mutagenesis as described above. Culture conditions E. coli B strain BL21(DE3) (Invitrogen catalog number C600003) was used in all experiments. Cells transformed with appropriate plasmids were grown from a single colony in Lysogeny broth (LB) (Miller) at 25 °C with orbital shaking at 250 rpm overnight. Overnight cultures were pelleted (3000 × g , 5 min, 4 °C), washed, and resuspended with one culture volume of LB before seeding subcultures at OD 600 = 0.05 in Erlenmeyer flasks with loose lids. Subcultures were grown for 4 h (25 °C, 250 rpm) to OD 600 ~ 0.4–0.6, induced with 0.4 mM IPTG for 1 h, then induced for 45 min with 0.2% l -rhamnose. Growth media were supplemented with ampicillin (100 μg mL −1 ) or trimethoprim (50 μg mL −1 ) as necessary. Western immunoblotting, imaging and quantitation Proteins were separated by SDS-PAGE on 8–16% Tris-glycine gels (Invitrogen) and transferred to nitrocellulose membranes using an iBlotII (Life Technologies). Immunoblot buffer [Odyssey Blocking Buffer (Licor) diluted by half with PBS and supplemented with 0.01% Tween20] was used for all blocking and antibody/antisera incubations, PBS + 0.01% Tween20 (PBST) for initial washes, and PBS for final washes. Monoclonal mouse anti-StrepII and anti-His antibodies were obtained from Qiagen (catalog number 34850) and Genscript (catalog number A00186), respectively. Polyclonal rabbit antisera raised against EspP β-barrel and BamA C-terminal peptides have been described previously [30] . A polyclonal rabbit antiserum was also generated against a peptide derived from the N terminus of the EspP β-barrel domain (NH 2 -NLNKRMGDLRDINGEAGAWARC-COOH). Secondary antibodies [goat anti-mouse 800CW (IRDye catalog number 926–32210) and goat anti-rabbit 680LT (IRDye catalog number 926–68021)] were obtained from Licor. Membranes for quantitation were blocked for 1 h, incubated with anti-StrepII (1:5000 dilution) for 1 h, washed (3 × 5 min with PBST), incubated with goat anti-mouse 800CW (1:5000 dilution) for 1 h, washed (3 × 5 min with PBST, 2 × 5 min PBS), and air dried. The membranes were then scanned using an Amersham Typhoon 5 imager (GE Healthcare) with a 785 nm laser, IRlong 825BP30 filter, and PMT set at 700 V. Pixel intensities of detected proteins were measured using Fiji software (v2.0.0-rc-68/1.52 g). Within-lane values were used to calculate percent disulfide-bond formation [( MBP−76 EspP- His BamA/(free MBP−76 EspP + MBP−76 EspP- His BamA) × 100]. Otherwise, membranes for single- or duplex-immunoblots were typically incubated overnight with primary antibodies/antisera and for 2 h with secondary antibodies. Dried membranes were imaged with an Odyssey infrared imager (Licor, model 9120) or a Typhoon 5 imager using maximum quality and resolution settings. Uncropped images of all blots are included in the Source Data file. Cell surface protease digestions and arrest-release assembly To monitor the surface exposure of the MBP−76 EspP linker or the protease sensitivity of BamA loop 6, 1 mL samples of induced bacterial subcultures were aliquoted into 1.5 mL tubes on ice. Cells were pelleted (10,000 × g , 2 min, 4 °C), resuspended in 0.5 mL PBS, and incubated on ice for 20 min (unless otherwise indicated) with 200 μg mL −1 Proteinase K (PK) or equivalent volume of PK buffer (5 mM CaCl 2 , 50 mM Tris-HCL pH 8) for the mock-treated control. For TEV digestions, cells were resuspended in M9 medium with 2 mM DTT and incubated at 25 °C for 2 h with 50 μg mL −1 TEV protease (hyperactive S219V mutant, obtained from Dr. Susan Buchanan). To observe the completion of β-barrel assembly following the release of MBP, cells were resuspended in PBS at 25 °C and incubated with 200 μg mL −1 PK [25 °C, 350 rpm, in a Thermomixer (Eppendorf)] for 0.5, 2, 10 and 30 min. Cells were then pelleted (10,000 × g , 20 s, 4 °C), resuspended in 0.5 mL PBS, and incubated with 4 mM PMSF and 10% (v/v) TCA on ice for 10 min to inhibit PK and precipitate proteins. TCA precipitates were pelleted (20,817 × g , 10 min, 4 °C), washed with 0.6 mL acetone, pelleted again, and air dried at 37 °C for 15 min. Dried precipitates were resuspended with 2x SDS protein gel loading solution (Quality Biological) in a volume normalised to the final OD 600 reading (volume, μL = OD 600 × 200) and heated at 99 °C for 15 min. Disulfide-bond formation assay To observe site-specific intermolecular protein-protein interactions, 1 mL samples of induced subculture cells were aliquoted into 1.5 mL tubes on ice, pelleted (10,000 × g , 2 min, 4 °C), and resuspended in 1 mL PBS. Cells were incubated with the thiol-specific oxidiser 4,4′-dipyridyl disulfide (4-DPS) at a final concentration of 0.2 mM (or an equivalent volume of ethanol for mock-treated controls) and incubated on ice for 30 min. Cells were then pelleted (10,000 × g , 2 min, 4 °C), resuspended in 0.5 mL PBS, and mixed with TCA to precipitate proteins as described above. To monitor the kinetics of intermolecular disulfide-bond formation, 5 mL samples of induced subculture were aliquoted into 50 mL tubes on ice, pelleted (3000 × g , 4 min, 4 °C), and washed with 10 mL PBS. Cells were then resuspended in 5 mL PBS and incubated with 0.2 mM 4-DPS or ethanol (mock-treated) for 0, 2, 5, 15, 30, 60 and 90 min. At each time point 0.4 mL aliquots were dispensed into 1.5 ml tubes pre-loaded with PMSF and TCA for instant protein precipitation. TCA precipitates were washed and mixed with 2x SDS protein gel loading solution as described above. Control samples were reduced with 150 mM dithiothreitol (DTT) during heating. Release of assembly arrest and disulfide-bond reduction To restart β-barrel assembly following the release of MBP and the reduction of MBP−76 EspP- His BamA inter-barrel disulfide-bonds, 20 mL samples of induced subculture were aliquoted into 50 mL tubes on ice and pelleted (3000 × g , 5 min, 4 °C). Cells were washed with 40 mL PBS, pelleted (4000 × g , 6 min, 4 °C), and resuspended in 10 mL PBS. Cell aliquots (0.5 mL) were placed into 1.5 mL tubes, incubated with 0.2 mM 4-DPS for 30 min on ice, pelleted (10,000 × g , 2 min, 4 °C), and resuspended in 0.5 mL PBS. Cells were then incubated with either 200 μg mL −1 PK or PK buffer (mock digest) for 30 min on ice, washed with 1 mL PBS, and resuspended in 0.5 mL PBS (containing 1 mM PMSF) pre-warmed to 25 °C. Cells were then incubated in a Thermomixer (25 °C, 350 rpm) either in 50 mM HEPES pH 7 containing 150 mM DTT or without DTT (mock-treated) for 0.5, 2, 5 and 15 min. All samples were TCA precipitated on ice and prepared for SDS-PAGE as above. Gel mobility-shift assay To observe hybrid-barrel conformational states, cysteine pairs were oxidised as described above. Cells were then resuspended in BugBuster Master Mix (EMD Millipore) containing EDTA-free SigmaFast protease inhibitor (Sigma-Aldrich) (volume, μL = OD 600 × 100) and lysed on ice for 3 min. Aliquots (30 μL) of lysates were mixed with 10 μL 2x SDS protein gel loading solution to bring the final SDS concentration to 1%. Samples were either maintained on ice or heated to 99 °C for 10 min. Proteins were then resolved by ‘cold’ SDS-PAGE (i.e., by packing gel tanks in ice and running the gels in a 4 °C room) and transferred to nitrocellulose for immunoblotting as described above.